Dehydrogenation of anhydrous methanol at room temperature byo-aminophenol-based photocatalysts Dehydrogenation of anhydrous methanol is of great importance, given its ubiquity as an intermediate for the production of a large number of industrial chemicals. Since dehydrogenation of methanol is an endothermic reaction, heterogeneous or homogeneous precious-metal-based catalysts and high temperatures are usually required for this reaction to proceed. Here we report the photochemical dehydrogenation of anhydrous methanol at room temperature catalysed by o -aminophenol (apH 2 ), o -aminophenolate (apH − ) and the non-precious metal complex trans -[Fe II (apH) 2 (MeOH) 2 ]. Under excitation at 289±10 nm and in the absence of additional photosensitizers, these photocatalysts generate hydrogen and formaldehyde from anhydrous methanol with external quantum yields of 2.9±0.15%, 3.7±0.19% and 4.8±0.24%, respectively, which are the highest values reported so far to the best of our knowledge. Mechanistic investigations reveal that the photo-induced formation of hydrogen radicals triggers the reaction. Molecular hydrogen (H 2 ) is one of the most promising energy sources of the future [1] , [2] , [3] , [4] , [5] , [6] . As gaseous H 2 is difficult to handle and store, hydrogen storage materials have been the subject of intensive investigation in recent years [7] , [8] , [9] . Among a number of materials, methanol (MeOH) represents one of the most fascinating hydrogen carriers [10] , [11] , [12] , [13] , [14] , [15] , which is used in fuel cells [16] , [17] , [18] , [19] due to its high-gravimetric H 2 content (12.6 wt% H 2 ). Since the generation of H 2 from MeOH is an endothermic reaction, both dehydrogenation catalysts and high temperatures are usually required for this reaction to proceed, and several heterogeneous [20] and homogeneous [21] , [22] , [23] , [24] , [25] , [26] catalyst systems have been investigated in this context [27] , [28] . Homogeneous catalytic systems for the dehydrogenation of MeOH can be classified into three types: (1) thermal dehydrogenation catalysts for hydrous MeOH (MeOH reforming), (2) thermal dehydrogenation catalysts for anhydrous MeOH and (3) photochemical dehydrogenation catalysts for anhydrous MeOH. Beller et al . reported that the use of [Ru II (H)Cl(PNP)] (PNP=HN(C 2 H 4 P i -Pr 2 ) 2 ) [21] and of the non-precious metal complex [Fe II (H)(BH 4 )(PNP)] [22] allowed a dehydrogenation of the MeOH/H 2 O mixture to CO 2 (or CO 3 2− ) at 91 °C. Other examples were reported by Grützmacher and co-workers [23] , and Crabtree and co-workers [29] , who demonstrated that the dehydrogenation of MeOH is catalysed at 91 °C by [Ru II (H)(1,4-bis(5H-dibenzo[a,d]cyclohepten-5-yl)-1,4-diazabuta-1,3-diene)] − or [Ir I (CO) 2 ( N,N -dimethylheterocyclic carbene) 2 ] + complexes, respectively. Milstein and co-workers [26] observed the formation of H 2 from mixtures of MeOH/H 2 O/THF in the presence of [Ru II (H)(Cl)(CO)(BPy- t PNN)] (BPy- t PNN=6-di- tert -butylphosphinomethyl-2,2′-bipyridine) at 60 °C. Conversely, Saito et al . and Shinoda et al . [30] , [31] , [32] , [33] reported several Ru-complexes as thermal dehydrogenation catalysts for anhydrous MeOH, which operate at 64–79 °C (TONs H2 =8–34; TOF H2 =0.94–1.23 h −1 ). One promising strategy to lower the undesirably high reaction temperatures are photochemical reactions [34] , [35] , [36] , [37] , [38] , [39] . Photochemical dehydrogenations of anhydrous MeOH should be highly attractive for two reasons: anhydrous HCHO, produced form anhydrous MeOH, is an important intermediate for the production of a large number of industrial chemicals [40] , and the lack of effective catalysts for the removal of H 2 O from aqueous HCHO renders this process relatively cost intensive. 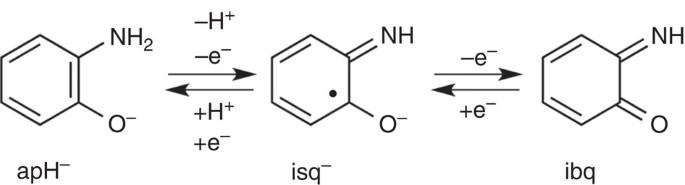Figure 1: Electron- and proton-transfer properties of apH−. On removal of one proton and one-electron,o-aminophenolate (apH−) reversibly affordso-iminosemiquinonate (isq−), which is reversibly transferred intoo-iminobenzoquinone (ibq) on a further one-electron oxidation. To the best of our knowledge, only six homogenous photocatalysts or catalyst precursors for the photochemical dehydrogenation of anhydrous MeOH have been reported during the past three decades ( Supplementary Table 1 ) [34] , [35] , [36] , [37] , [38] , [39] . Saito and co-workers [36] , [37] , [38] , [39] reported the dehydrogenation of anhydrous MeOH under concomitant formation of H 2 at 64–65 °C, using Rh, Pd and Ir-based precious metal catalysts. The reaction could also be carried out at 20 °C using cis -[Rh I 2 (Cl) 2 (CO) 2 (dpm) 2 ] (dpm=bis(diphenylphosphino)methane), albeit that the presence of acetone as an additional photosensitizer was required, which led to the formation of considerable amounts of by-products, such as HOC(CH 3 ) 2 C(CH 3 ) 2 OH [36] . These pioneering studies motivated us to develop a new catalytic platform for the dehydrogenation of anhydrous MeOH at ambient temperature, which requires neither precious metals nor additional photosensitizers. We have recently reported that [Fe II (opda) 3 ] 2+ (opda= o -phenylenediamine) is able to photochemically generate H 2 in tetrahydrofuran [41] . In this reaction, opda does not only act as a chelating ligand via the two amino groups, but also as a multi-electron and proton-pooling site for the photochemical generation of H 2 at ambient temperature. We proposed that H 2 is released as a result of the photochemical activation of the N–H bonds in the amino moieties of opda, accompanied by an oxidation to afford the oxidized semi-benzoquinodiimine or o -benzoquinodiimine species. In contrast to the homoleptic coordination of opda via two amino groups, the corresponding o -aminophenolato ligand (apH − ) displays a heteroleptic coordination pattern via one amino and the deprotonated hydroxyl group, which should facilitate the transfer of two electrons and one proton ( Fig. 1 ) [42] , [43] , [44] , [45] , [46] . Pino and co-workers [47] have reported the 1 π-π*-initiated photochemical activation of the O–H bond of o -aminophenol (apH 2 ) in the gas phase. This characteristic reactivity, which occurs on the picosecond timescale in the gas phase at 65–90 °C, has recently been labelled ‘excited state hydrogen detachment (ESHD)’. However, there is a considerable gap between the ESHD of aromatic amines and alcohols and the photochemical hydrogen evolution reaction (PHER) of [Fe II (opda) 3 ] 2+ , because the generation of H 2 has not yet been reported for the ESHD system. Figure 1: Electron- and proton-transfer properties of apH − . On removal of one proton and one-electron, o -aminophenolate (apH − ) reversibly affords o -iminosemiquinonate (isq − ), which is reversibly transferred into o -iminobenzoquinone (ibq) on a further one-electron oxidation. Full size image Recently, successful examples on the elucidation of electron- and proton-transfer properties of transition metal complexes of apH − , together with the characterization of corresponding complexes with o -iminosemiquinonate (isq − ) have been reported, and these studies are currently under extensive investigation as models for non-haem-type iron dioxygenase [42] , [43] , [44] , [45] , [46] . In contrast to these sophisticated examples for the reactivity of apH 2 derivatives, which proceed under the exclusion of light, examples on photochemical reactions still remain elusive. Here we report the photochemical dehydrogenation of anhydrous MeOH at room temperature catalysed by apH 2 , apH − and the non-precious metal complex trans -[Fe II (apH) 2 (MeOH) 2 ] ( 1 ). These photocatalysts promote the PHER from MeOH in the absence of additional photosensitizers, and generated H 2 and HCHO with the highest external quantum yields ( Φ H2 ) reported so far. Mechanistic investigations revealed that the photo-induced formation of hydrogen radicals triggers the PHERs. Moreover, the complexation between Fe II and apH − facilitates the photochemical generation of H 2 at longer wavelengths. The observed PHER activity promises potential for these compounds to serve as a new photocatalyst platform. 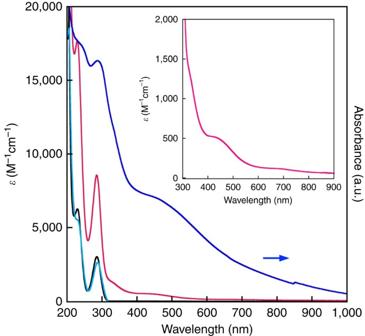Figure 2: Ultraviolet–visible–near infrared spectra of apH2-based photocatalysts in MeOH. [apH2(black line)]=[apH−(turquoise line)]=2 mM; [1(magenta line)]=1.35 mM. The generation of apH−was accomplishedin situby the treatment of apH2with TBAOH. The solid-state spectrum of1(KBr disk, blue line) is shown for comparison. The inset shows a magnification for the 300–900 nm region of the solution spectrum of1. PHERs of MeOH by apH 2 and apH − Figure 2 shows the ultraviolet–visible–near infrared spectra of apH 2 (2.00 mM) and apH − (2.00 mM), whereby the latter was generated in situ by the treatment of apH 2 with one equivalent of tetra- n -butyl ammonium hydroxide (TBAOH). For both apH 2 and apH − , two absorptions were observed at λ max ( ɛ /M −1 cm −1 )=230 (6,260) and 285 nm (3,020), as well as at 230 (5,540) and 288 nm (2,630), respectively ( Supplementary Table 2 ). These bands were assigned to two π−π* transitions [47] , and the observed similarity of the spectral profiles indicates a negligible effect of the deprotonation of apH 2 on the π−π* transitions. Figure 2: Ultraviolet–visible–near infrared spectra of apH 2 -based photocatalysts in MeOH. [apH 2 (black line)]=[apH − (turquoise line)]=2 mM; [ 1 (magenta line)]=1.35 mM. The generation of apH − was accomplished in situ by the treatment of apH 2 with TBAOH. The solid-state spectrum of 1 (KBr disk, blue line) is shown for comparison. The inset shows a magnification for the 300–900 nm region of the solution spectrum of 1 . Full size image MeOH solutions of both apH 2 and apH − did not exhibit any signs of gas evolution under the exclusion of light. However, the photoirradiation (289±10 nm; 3.2 mW Hg–Xe lamp) of a MeOH solution of apH 2 induced the evolution of gas, and a gas chromatography (GC) analysis of a gaseous sample taken from the headspace of the reaction vessel allowed the detection of H 2 ( Supplementary Fig. 1 ). After 5 h of photoirradiation, 4.1±0.21 equiv. of H 2 per molecule of apH 2 ( Φ H2 =2.9±0.15%) were obtained ( Fig. 3 , Table 1 , and Supplementary Fig. 2 ), while up to 6.5±0.33 equiv. H 2 per molecule of apH 2 were obtained after 24 h of photoirradiation ( Supplementary Fig. 3 ), suggesting that the reaction is not stoichiometric, but catalytic. Deprotonated apH − exhibits a similar PHER activity ( Φ H2 =3.7±0.19%) on irradiation at 289±10 nm. Control reactions, using neat MeOH under otherwise identical conditions, did not exhibit any PHER activity. Considering these PHER results and the aforementioned absorption spectra, it is feasible to assume that the π−π* excitation of apH 2 and apH − initiates the PHERs. 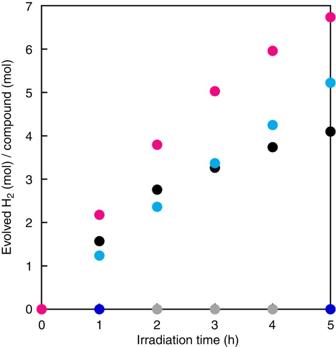Figure 3: H2evolution from MeOH solutions of apH2-based photocatalysts. Mols of evolved H2per mols of catalyst as a function of PHER time for MeOH solutions of apH2(2 mM; black circles), apH−(2 mM; turquoise circles),1(1 mM; magenta circles), and FeII(ClO4)2·6H2O (1 mM; blue circles), together with pure MeOH (grey circles). Irradiation wavelength, 289±10 nm (3.2 mW). Estimated relative s.d., 5%. Figure 3: H 2 evolution from MeOH solutions of apH 2 -based photocatalysts. Mols of evolved H 2 per mols of catalyst as a function of PHER time for MeOH solutions of apH 2 (2 mM; black circles), apH − (2 mM; turquoise circles), 1 (1 mM; magenta circles), and Fe II (ClO 4 ) 2 ·6H 2 O (1 mM; blue circles), together with pure MeOH (grey circles). Irradiation wavelength, 289±10 nm (3.2 mW). Estimated relative s.d., 5%. Full size image Table 1 PHER products from the photochemical reactions of apH 2 -based photocatalysts * . Full size table In general, oxidation of anhydrous MeOH should afford oxidized species such as formaldehyde (HCHO) [37] , [38] , [39] and methyl formate (HCO 2 Me) [31] , [33] . In the case that small amount of H 2 O contaminates, formic acid (HCO 2 H) [37] , [38] , [39] and CO 2 [21] , [22] are also produced as minor products. After PHER of apH 2 (5 h), a high-performance liquid chromatography (HPLC) analysis revealed that 3.3±0.08 equiv. of HCHO were generated per molecule of apH 2 ( Table 1 and Supplementary Fig. 4a ). Taking the experimental errors (3 standard deviation (s.d.)) into account, the difference between the quantities of the two products is statistically not significant, corroborating the photochemical dehydrogenation of MeOH. Furthermore, prolonged PHER (24 h) afforded a small amount of HCO 2 H and/or HCO 2 Me (HCO 2 H/HCO 2 Me), which was produced from dehydrogenation of HCHO in the presence of trace amounts of residual H 2 O, in addition to H 2 and HCHO ( Table 1 and Supplementary Fig. 4b ). This reaction thus represents the first example of an organophotocatalyst promoting the photochemical dehydrogenation of MeOH to generate H 2 . In particular, the external quantum yields (apH 2 : Φ H2 =2.9±0.15; apH − : Φ H2 =3.7±0.19%) are the highest value in those of previously reported molecular photocatalysts (for more details, see Supplementary Table 1 ) [25] , [30] , [31] , [32] . PHERs of MeOH by trans -[Fe II (apH) 2 (MeOH) 2 ] (1) Mixing two equivalents of apH 2 and TBAOH with Fe II (ClO 4 ) 2 ·6H 2 O in MeOH under an atmosphere of N 2 afforded colourless crystals of 1 ( Supplementary Table 3 ). The molecular structure of 1 is shown in Fig. 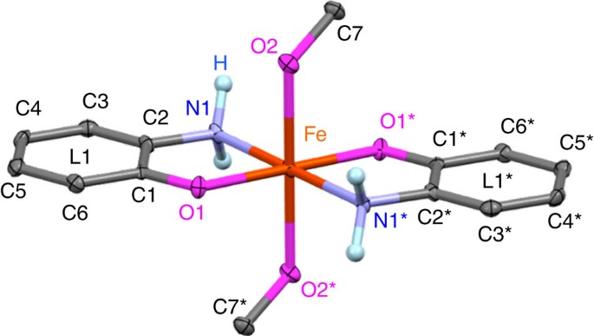Figure 4: Molecular structure of 1. Atomic displacement parameters set at 50% probability; colour code: C, dark grey; Fe, orange; N, light blue; O, magenta; ball-and-stick plots for N-bound hydrogen atoms (light blue), while all other hydrogen atoms are omitted for clarity. C1/C1*, C2/C2*, C3/C3*, C4/C4*, C5/C5*, C6/C6*, C7/C7*, N1/N1*, N2/N2*, O1/O1* and O2/O2* denote pairs of crystallographically equivalent atoms related by the symmetry operation 2–x, –y, 2–z. 4 , and selected bond distances are summarized in the Supplementary Table 4 . The structure of 1 is characterized by a pseudo-octahedral coordination geometry of the Fe atom, which is located on an inversion centre, and by two bidentate NO ligands that occupy the equatorial positions, while two monodentate O ligands reside on the apical positions. The two chelating ligands adopt a trans geometry, most likely to reduce steric repulsions [48] . The assignment of the two chelating ligands requires great care, as these could be apH − , isq − or o -iminobenzoquinone (ibq) ligands ( Fig. 1 ) [42] , [43] , [44] , [45] , [46] . In complex 1 , the observed C–N and C–O bond distances of 1.461(5) Å and 1.342(5) Å, respectively, suggest a single-bond character for these bonds [41] , [43] , [44] , [45] , [46] , [49] . Moreover, the observed C–C bond distances of 1.385–1.417(6) Å within the six-membered ring indicate high levels of aromaticity. While apH 2 contains one hydroxyl and two amino protons, which can be deprotonated by TBAOH (1 equiv.) to give monoanionic C 6 H 4 NOH 2 − , previous reports on Fe(II) complexes of apH − have shown that it is possible to deprotonate the hydroxyl proton in apH 2 selectively [43] , [44] , [45] , [46] . As the Fe–O1 (2.048(3) Å) and Fe–N1 (2.214(4) Å) bond distances in 1 are comparable to those in these examples (Fe–O: 1.931–1.994(2) Å; Fe–N: 2.212–2.299(7) Å), the structure of the chelating ligands should be commensurate with that of apH − . Furthermore, the selective deprotonation of the hydroxyl proton was consistent with typical p K a values for aromatic amines (for example, p K a aniline=30.6) [50] and alcohols (for example, p K a phenol=18.0) [51] . While the observed Fe–O2 bond distance (2.229(3) Å) is comparable to those of typical Fe II –HOMe bonds (2.205(16) Å) [52] , it is substantially longer than typical Fe II –OMe bonds (1.782(3) Å) [53] . Accordingly, the axial ligands should be MeOH ligands. Moreover, the Fe–N1, Fe–O2 and Fe–O1 bond distances of 2.214(4) Å, 2.229(3) Å and 2.048(3) Å, respectively, suggest the presence of a high-spin Fe II centre [43] , [44] , [45] , [46] . These observations, in their entirety, suggest that 1 adopts a structure that is consistent with trans -[Fe II (apH) 2 (MeOH) 2 ]. Figure 4: Molecular structure of 1. Atomic displacement parameters set at 50% probability; colour code: C, dark grey; Fe, orange; N, light blue; O, magenta; ball-and-stick plots for N-bound hydrogen atoms (light blue), while all other hydrogen atoms are omitted for clarity. C1/C1*, C2/C2*, C3/C3*, C4/C4*, C5/C5*, C6/C6*, C7/C7*, N1/N1*, N2/N2*, O1/O1* and O2/O2* denote pairs of crystallographically equivalent atoms related by the symmetry operation 2– x , – y , 2– z . Full size image It should be noted that the Fe–N1 bond distance (2.214(4) Å) in 1 is similar to those in [Fe II (opda) 3 ](ClO 4 ) 2 (2.204–2.234(2) Å), whereas the dihedral angle between the O1–Fe1–N1 and O1–C1–C2–N1 planes in 1 (1.06°) is relatively small compared with those in [Fe II (opda) 3 ](ClO 4 ) 2 (35.90, 38.17 and 44.15°) [41] . The high levels of planarity in the five-membered rings that contain the Fe II centre in 1 are indicative for the presence of interactions between the d -orbitals of Fe II and the π-orbitals of the apH − moieties via the p -orbitals on the O atom(s) [43] . It is also noteworthy that the observed differences with respect to the dihedral angles induce a substantially different coordination environment for the amino groups in 1 relative to those in [Fe II (opda) 3 ](ClO 4 ) 2 (ref. 41 ). The ultraviolet–visible–near infrared spectra of 1 (1.35 mM) in MeOH, as well as that of solid 1 (KBr disk) are shown in Fig. 2 . For 1 , four absorption bands were observed at λ max ( ɛ /(M −1 cm −1 ))=230 (17,690), 285 (8,550), 335 (1,210), 460 (480) and 680 nm (118). The two absorption bands at 230 and 285 nm, with relatively large molar extinction coefficients, are similar to those of apH 2 and apH − , and were therefore assigned to the transitions involving apH − -centred π−π* transitions [47] . The two bands at 335 nm and 460 nm, which were not observed for apH 2 and apH − , were tentatively assigned to charge transfer (CT) transitions between Fe(II) and the apH − ligands [45] , while the d–d transitions of the Fe(II) centre appeared as a shoulder band at 680 nm (118 M −1 cm −1 ). In the solid state, the absorption bands of 1 appeared at 235, 287, 335, 450 and 750 nm, similar to those of the MeOH solution, suggesting comparable structures in solution and in the solid state. As metal ions are known to interact with apH − and perturb its properties, the bis-( o -aminophenolato) Cu(II) analogue [Cu II (apH) 2 (H 2 O)] was synthesized and structurally characterized to assess possible effects of the presence of metal ions (see Supplementary Note 1 , as well as Supplementary Figs 5 and 6 , and Supplementary Table 2 ). Under an atmosphere of N 2 and under the exclusion of light, 1 is reasonably stable in MeOH ( Supplementary Fig. 7a ). In contrast, the corresponding Cu(II) complex exhibited a time-dependent spectral change under the same conditions, which is indicative of the formation of 2-aminophenoxazine-3-one (APX) ( Supplementary Figs 7b and 8 ). These results suggest a remarkable influence of the metal centre on the electron-donating ability of the apH − ligand. As the Cu complex proved to be unstable in MeOH, no PHER experiments were carried out on this complex. Figure 3 shows the amount of evolved H 2 as the result of the photoirradiation ( λ irr =289±10 nm; 3.2 mW Hg–Xe lamp; 5 h) of a MeOH solution of 1 (magenta circles). The MeOH solution of 1 also showed PHER activity, resulting in the formation of 6.7±0.34 (5 h) and 14.9±0.75 (24 h) mols of H 2 per mol of 1 , respectively ( Supplementary Fig. 3 ). In addition to H 2 and HCHO, prolonged PHER (24 h) also afforded small amounts of HCO 2 H/HCO 2 Me ( Table 1 ), while evidence for the formation of CO 2 was not observed. Control reactions under the same conditions, using a MeOH solution of Fe II (ClO 4 ) 2 ·6H 2 O did not show any PHER activity ( Fig. 3 and Supplementary Fig. 2 ). Moreover, a MeOH solution of Fe II (ClO 4 ) 2 ·6H 2 O containing 2 equiv. of opda generated only minor amounts of H 2 , indicating a lower activity of the opda complex of Fe(II) relative to that of 1 ( Supplementary Fig. 9 ). For the PHER of a MeOH solution of 1 , a Φ H2 value of 4.8±0.24% (5 h) was estimated. Considering these PHER results and the aforementioned absorption spectra, it is feasible to suggest that the photoexcitation of the apH − ligand in 1 initiates the PHER. Even when the PHER of 1 was carried out at 45 °C, no temperature dependence was observed, which in turn suggests that the photochemical process should be the rate-determining step of the PHER ( Supplementary Fig. 10 ). Interestingly, the photocatalytic activity on apH − was not suppressed even after the complexation with the Fe II centre, implying the possibility to tune the reactivity of the system via a variation of the metal ion. To determine the excitation that initiates the PHER of 1 in MeOH, we examined the correlation between the PHER performance and the wavelength of the irradiation source. Exposing a MeOH solution of 1 to photoirradiation at 460±10 nm ( ɛ 460 nm =483 M −1 cm −1 , 24 h) did not generate any H 2 . However, exposing a MeOH solution of 1 to photoirradiation at 350±10 nm (21.8 mW, ɛ 350 nm =932 M −1 cm −1 , 24 h) initiated PHER and resulted in the formation of 0.48±0.02 equiv. of H 2 with an estimated Φ H2 value of 0.019±0.001% ( Fig. 5 and Supplementary Fig. 11 ). Although the Φ H2 value for an irradiation at 350±10 nm (0.019±0.001%) is lower than that at 289±10 nm (4.8±0.24%), these results imply that the PHER may be driven by lower-energy light sources, given a suitable combination of apH − -type ligands and metal ions. 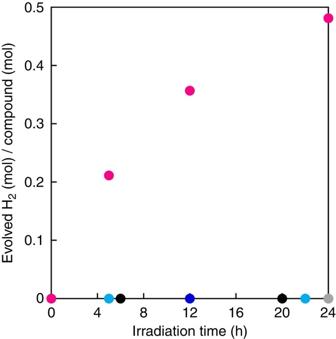Figure 5: H2evolution from a MeOH solution of 1. Mols of evolved H2per mol of catalyst as a function of PHER time for MeOH solutions of apH2(2 mM; black circles), apH−(2 mM; turquoise circles),1(1 mM; magenta circles) and FeII(ClO4)2·6H2O (1 mM; blue circles), together with pure MeOH (grey circles). Irradiation wavelength, 350±10 nm (21.8 mW). Estimated relative s.d., 5%. Figure 5: H 2 evolution from a MeOH solution of 1. Mols of evolved H 2 per mol of catalyst as a function of PHER time for MeOH solutions of apH 2 (2 mM; black circles), apH − (2 mM; turquoise circles), 1 (1 mM; magenta circles) and Fe II (ClO 4 ) 2 ·6H 2 O (1 mM; blue circles), together with pure MeOH (grey circles). Irradiation wavelength, 350±10 nm (21.8 mW). Estimated relative s.d., 5%. Full size image A reaction mechanism for the PHERs For the photochemical dehydrogenation of anhydrous MeOH, reports on detailed investigations regarding the mechanism on a molecular level remain scarce so far [35] , [36] , [37] , [38] , [39] . Therefore, we wanted to shed some light on the fundamental PHER mechanism that is operative in the MeOH solutions of apH 2 , apH − and 1 , and we were especially interested in the source of the evolved H 2 . In this system, it is pertinent to distinguish proton and electron sources according to: (i) the hydroxyl and methyl protons of MeOH, (ii) the aromatic protons of apH 2 , apH − and apH − in 1 , and (iii) the amino protons of apH 2 , apH − and apH − in 1 . Taking the amount of photochemically generated H 2 and HCHO into account ( Table 1 ), together with the small amounts of HCO 2 H/HCO 2 Me, it seems plausible to consider (i) as the most probable source of the evolved H 2 . To experimentally confirm this hypothesis, PHERs were carried out in MeOH- d 3 , and the evolved gas was analysed by GC at 77 K ( Fig. 6 ). For H 2 , D 2 and HD standards, retention times of 5.0 ( p -H 2 ), 6.3 ( o -H 2 ), 7.8 ( p -D 2 ), 8.4 ( o -D 2 ) and 6.4 min (HD) were observed ( Fig. 6a–c ). Photoirradiation of apH 2 in MeOH- d 3 at 289±10 nm afforded gas samples that exhibited a single peak with a retention time of 6.4 min. ( Fig. 6d ), suggesting the selective formation of HD under such PHER conditions. Clearly, the D atom in the evolved HD originates from an α -hydrogen of MeOH- d 3 , thus suggesting a C–H(D) bond cleavage during PHER. The PHER of apH − and 1 ( Fig. 6e,f ), as well as the photoirradiation of a MeOH- d 3 solution of 1 at 350±10 nm ( Fig. 6g ) furnished samples that displayed similar HD peaks in the GC analysis. These results confirm that the PHER of MeOH solutions of apH 2 , apH − and 1 generate H 2 from MeOH. 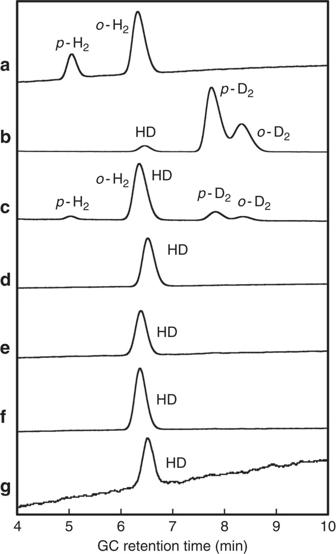Figure 6: GC analysis of the gaseous PHER products. GC profiles of (a) H2, (b) D2and HD generated by treatment of MeOH-d4(99.8%) with sodium metal, and (c) HD, H2and D2generated by the treatment of a mixed MeOH/MeOH-d4solution (v/v=1/1) with sodium metal; gas samples obtained from MeOH-d3(99.5%) solutions of (d) apH2, (e) apH−and (f)1after photoirradiation at 289±10 nm (3.2 mW, 24 h) and (g)1after photoirradiation at 350±10 nm (21.8 mW, 24 h); GC conditions: 8% KOH alumina column;T=77 K. Figure 6: GC analysis of the gaseous PHER products. GC profiles of ( a ) H 2 , ( b ) D 2 and HD generated by treatment of MeOH- d 4 (99.8%) with sodium metal, and ( c ) HD, H 2 and D 2 generated by the treatment of a mixed MeOH/MeOH- d 4 solution ( v / v =1/1) with sodium metal; gas samples obtained from MeOH- d 3 (99.5%) solutions of ( d ) apH 2 , ( e ) apH − and ( f ) 1 after photoirradiation at 289±10 nm (3.2 mW, 24 h) and ( g ) 1 after photoirradiation at 350±10 nm (21.8 mW, 24 h); GC conditions: 8% KOH alumina column; T =77 K. Full size image As apH 2 and apH − can promote one-proton and two-electron transfers, it is not surprising that these can generate electron(s), hydrogen radical(s) or a hydride ( Fig. 1 ). To gain a better mechanistic understanding of the observed PHERs, photochemical reactions were carried out in the presence of 2-methylpropane-2-thiol ( t -BuSH), which is able to act as a hydrogen radical scavenger on account of the relatively low-bond dissociation energy of the S–H bond, resulting in the formation of di- tert -butyl disulfide ( t -Bu 2 S 2 ) [54] . The 1 H NMR spectrum of t -BuSH prior to photoirradiation at 289±10 nm (24 h) in MeOH- d 4 is shown in Fig. 7a . A singlet peak was observed at δ =1.40 p.p.m. and assigned to the protons of the t -Bu group. After photoirradiation, no considerable change was observed in the spectrum ( Supplementary Fig. 12 ), which is consistent with the absence of an absorption ∼ 289 nm ( Supplementary Fig. 13 ). The 1 H NMR and ultraviolet–visible spectra of t -Bu 2 S 2 in MeOH- d 4 and MeOH are shown in Fig. 7b and Supplementary Fig. 13 , respectively. In MeOH- d 4 , the 1 H NMR spectrum of t -Bu 2 S 2 exhibits a singlet resonance at 1.29 p.p.m., while the ultraviolet–visible spectrum shows an absorption ∼ 289 nm in MeOH ( Supplementary Fig. 13 ). After photoirradiation of a MeOH- d 4 solution of t -Bu 2 S 2 at 289±10 nm (5 h), major singlet peaks emerged at 1.71, 1.40, 1.29 and 0.88 p.p.m. together with several minor peaks, which demonstrates the photochemical reactivity of t -Bu 2 S 2 ( Fig. 7c ). These resonances are thus indicative of the in situ formation of t -Bu 2 S 2 and the reaction products from its photochemical decomposition. 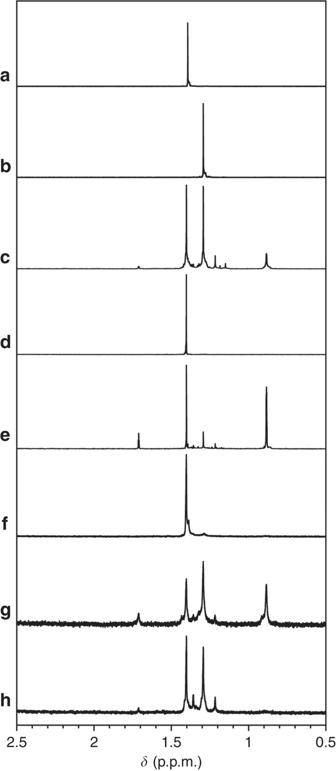Figure 7:1H NMR spectra of PHER products in the presence of hydrogen radical scavengers. 1H NMR spectra (MeOH-d4) of (a)t-BuSH, (b)t-Bu2S2, (c)t-Bu2S2after photoirradiation at 289±10 nm (5 h), (d)t-BuSH with apH2, (e)t-BuSH with apH2after photoirradiation at 289±10 nm (5 h), (f)t-BuSH with1, (g)t-BuSH with1after photoirradiation at 289±10 nm (5 h) and (h)t-BuSH with1after photoirradiation at 350±10 nm (24 h). Figure 7: 1 H NMR spectra of PHER products in the presence of hydrogen radical scavengers. 1 H NMR spectra (MeOH- d 4 ) of ( a ) t -BuSH, ( b ) t -Bu 2 S 2 , ( c ) t -Bu 2 S 2 after photoirradiation at 289±10 nm (5 h), ( d ) t -BuSH with apH 2 , ( e ) t -BuSH with apH 2 after photoirradiation at 289±10 nm (5 h), ( f ) t -BuSH with 1 , ( g ) t -BuSH with 1 after photoirradiation at 289±10 nm (5 h) and ( h ) t -BuSH with 1 after photoirradiation at 350±10 nm (24 h). Full size image The 1 H NMR spectrum of a mixture of t -BuSH and apH 2 in MeOH- d 4 ( Fig. 7d and Supplementary Fig. 14 ) displays a peak at 1.40 p.p.m., which is comparable to the resonances of pure t -BuSH in MeOH- d 4 ( Fig. 7a ), thus suggesting negligible interaction between apH 2 and t -BuSH in the ground state. After photoirradiation of this solution at 289±10 nm (5 h), new singlet peaks emerged at 1.71, 1.29, 1.22 and 0.88 p.p.m. ( Fig. 7e ). The new peaks are identical to those obtained for photoreacted t -Bu 2 S 2 ( Fig. 7c ), suggesting the formation of t -Bu 2 S 2 during the photoreaction of apH 2 and t -BuSH. Similar experiments were also carried out for 1 , but the 1 H NMR spectrum of t -BuSH in the presence of 1 ( Fig. 7a,f , and Supplementary Fig. 15 ) did not indicate any significant interaction between t -BuSH and paramagnetic 1 in the ground state. After photoirradiation of this solution at 289±10 nm (5 h), new singlet peaks were observed at 1.71, 1.29, 1.22 and 0.88 p.p.m. ( Fig. 7g ). These peaks are comparable to those of the photoirradiation product obtained from t -BuSH and apH 2 ( Fig. 7e ), and these results thus suggest the formation of t -Bu 2 S 2 from t -BuSH in the presence of 1 . At this point, it should be beneficial to consider possible formation mechanisms for the formation of t -Bu 2 S 2 from t -BuSH. One possibility is the oxidation of t -BuSH by apH 2 in the excited state, while another is the generation of hydrogen radicals from photoirradiated apH 2 , followed by the abstraction of a hydrogen radical from t -BuSH. On excitation at 285 nm in MeOH, apH 2 exhibits an emission peak at 342 nm ( Supplementary Fig. 16a ). This emission was tentatively assigned to the 1 π–π* excited state, which was not quenched by t -BuSH. Therefore, the generation of a hydrogen radical from an alternative excited path represents a more likely mechanism compared with an electron transfer via the 1 π–π* excited state. Similar to the case of apH 2 , the emission peak of 1 in MeOH was not influenced by the presence of t -BuSH on excitation at 285 nm ( Supplementary Fig. 16b ). This result suggests that the PHER of 1 does not include the oxidation of t -BuSH by the excited state of 1 , but the generation of a hydrogen radical from 1 . Furthermore, the characteristic singlet peak for t -Bu 2 S 2 at 1.29 p.p.m. was observed after photoirradiation of 1 at 350±10 nm (24 h; Fig. 7h ). These results suggest that the pathway for the generation of hydrogen radials is also included in the excitation of 1 at 350±10 nm, similarly to the excitation of 1 and apH 2 at 289±10 nm. The photoirradiation of 1 in MeOH at 350±10 nm in the presence of 3-carbamyl-1-methylpyridinium chloride (NADCl), which is an electron or hydride scavenger [55] , [56] , revealed no considerable change in the 1 H NMR spectra prior and posterior to the photoreaction ( Supplementary Fig. 17 ). These results indicate that the photoreaction of 1 at 350±10 nm does not include any electron transfer or generation of hydrides, and these are thus consistent with a mechanism based on hydrogen radicals (for a plausible reaction mechanism in the presence of t -BuSH, see Supplementary Fig. 18 ). In general, hydrogen can be generated from MeOH using an electron donor, a hydrogen radical or a hydride. Reactions between MeOH- d 3 and sodium metal (electron donor) or NaBH 4 (hydride donor) showed that under these conditions, H 2 was produced selectively (equations 1 and 2, Fig. 6a–c , and Supplementary Fig. 19 ). In contrast, the formation of HD was negligible, as the o -H 2 / p -H 2 peak area ratio was almost identical to that of the H 2 standard ( Supplementary Table 5 ). Hydrogen radicals have previously been reported to react with the α -hydrogen atoms of MeOH to produce H 2 and the corresponding · CH 2 OH radical (equation 3) [57] . The · CH 2 OH radical is a good reducing agent and able to react with electron acceptors (EA) such as Fe(III) or Co(III), which affords HCHO as the oxidized species (equation 4). For apH 2 , proton- and electron-transfer properties should be expected, and apH 2 should thus be able to donate electrons, hydrides and/or hydrogen radicals. The ability to photochemically generate hydrogen radicals from the hydroxyl protons has already been reported for apH 2 (ref. 47 ). As previously mentioned, we confirmed that PHERs of MeOH- d 3 solutions of apH 2 , apH − and 1 selectively generate HD ( Fig. 6 ), which suggests a selective abstraction of the α -hydrogen atoms from MeOH. Actually, the generation of hydrogen radicals was confirmed in the photochemical reactions of apH 2 and 1 in the presence of the scavengers ( Fig. 7 ). Consequently, all PHERs should be initiated by the generation of a hydrogen radical. 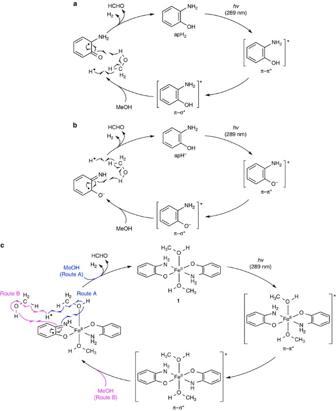Figure 8: Plausible PHER mechanisms. Reaction cycles catalysed by (a) apH2, (b) apH−and (c)1upon irradiation at 289±10 nm. Figure 8a shows a plausible mechanism for the PHER involving apH 2 . It seems reasonable to assume that PHER (289±10 nm) proceeds via the initial photochemical generation of hydrogen radicals from the hydroxyl moieties of apH 2 . Subsequently, H 2 and HCHO should be formed by the selective abstraction of α -hydrogen atoms from MeOH ( Fig. 6 ). The additional oxidation products (HCO 2 H/HCO 2 Me) would then be generated from the dehydrogenation of HCHO or from the dehydrogenation of HCHO in the presence of residual trace amounts of water. Figure 8: Plausible PHER mechanisms. Reaction cycles catalysed by ( a ) apH 2 , ( b ) apH − and ( c ) 1 upon irradiation at 289±10 nm. Full size image In the case of apH − , a hydroxyl proton is not present, and therefore, O–H bond cleavage in apH − should not occur during PHER. Previous studies on aromatic amines, such as aniline and opda, revealed characteristic photoreactions, which are initiated by the π−π* excitation through the 3 s Rydberg states of the nitrogen atom in the amino group [58] , [59] , [60] . Eventually, the N–H σ -bonds in these amino moieties are photochemically activated to generate hydrogen radicals via the π−π*/π− σ * conical intersection in these reactions, similar to the case of apH 2 (refs 61 , 62 ). The formation of a hydrogen radical and isq − may be possible from the homolytic cleavage of an N–H bond in the π− σ * exited state from a π−π* excitation ( Fig. 8b ), and subsequent reactions indicate the generation of H 2 and HCHO, similar to the case of apH 2 . Furthermore, complex 1 , containing apH − ligands, should also generate hydrogen radicals from the homolysis of an N–H bond in the apH − moiety under photoirradiation conditions (289±10 nm; Fig. 8c ). In the plausible mechanism for 1 , the MeOH molecule coordinated to the Fe(II) centre and/or that not directly bound to the Fe(II) centre may be included in the reaction as described in routes A and B ( Fig. 8c ). Remarkably, the complexation of apH − with Fe(II) does not inhibit its PHER activity. It should also be noted here that the PHER proceeding via excitations including π−π* transitions show higher Φ H2 values (4.8±0.24%) relative to CT excitations (0.019±0.001%). In this paper, we report the first examples for the photocatalytic dehydrogenation of anhydrous MeOH at room temperature, using apH 2 , apH − and an Fe(II) complex of apH − ( 1 ) as photocatalysts. These photocatalysts promote the PHER from MeOH in the absence of additional photosensitizers, and generate hydrogen and formaldehyde. For these PHERs, Φ H2 values based on the amount of generated H 2 , HCHO and HCO 2 H/HCO 2 Me were estimated using defined excitations at 289±10 or 350±10 nm. The observed PHER activity and the comparable Φ H2 values of apH 2 and apH − promise potential for these compounds as a new organophotocatalyst platform. Furthermore, 1 demonstrated a comparable photochemical reactivity and Φ H2 value relative to apH − , despite of the presence of a paramagnetic Fe(II) centre. The PHER activity on photoexcitation of the CT band of 1 suggested that the complexation between Fe II and apH − allows access to unprecedented photoreactivity that is able to realize the photochemical generation of H 2 at longer wavelengths compared with apH 2 and apH − . The central issues to be addressed in the immediate future concern improvements of the catalytic activity and the use of visible light as a driving force. These topics are currently under investigation in our laboratory, using various combinations of metal ions with apH − -type ligands and extended π-systems. General procedures Unless noted otherwise, all synthetic operations and measurements were carried out under an atmosphere of N 2 using Schlenk-line techniques. Fe II (ClO 4 ) 2 ·6H 2 O, Cu II (OAc) 2 ·H 2 O (OAc=acetate), HCO 2 H, acetic acid (AcOH), ammonium acetate (NH 4 OAc), acetyl acetone, calcium oxide (CaO) and H 2 SO 4 were purchased from Wako Pure Chemical Industries (Japan). Dehydrated MeOH, dichloromethane (CH 2 Cl 2 ) and MeOH- d 4 were purchased from Kanto Chemical Co. Inc. (Japan). TBAOH in MeOH (37%), which was used after the removal of MeOH, an aqueous solution of HCHO (37%), t -BuSH, t -Bu 2 S 2 , NADCl and apH 2 were purchased from Tokyo Chemical Industry Co. Ltd. (Japan). Prior to use, apH 2 was washed with CH 2 Cl 2 and dried in vacuo for several minutes, while t -BuSH was used after stirring with CaO for 12 h, followed by distillation. MeOH- d 3 was purchased from Sigma-Aldrich. APX was prepared according to a reported procedure [63] . All solvents that were used under anaerobic conditions were thoroughly degassed by at least five freeze–pump–thaw cycles immediately prior to use. Although we did not experience any difficulties with perchlorate salts, these should be regarded as potentially explosive, and therefore handled with utmost care. trans -[Fe II (apH) 2 (MeOH) 2 ] (1) A colourless MeOH solution (5 ml) of apH 2 (144 mg, 1.31 mmol) and TBAOH (340 mg, 1.31 mmol) was slowly deposited onto an aqua-blue MeOH (5 ml) solution of Fe II (ClO 4 ) 2 ·6H 2 O (240 mg, 0.661 mmol) under an atmosphere of N 2 . After leaving the solution to stand at 3 °C for a period of 5 days, colourless crystals of 1 , suitable for X-ray crystallographic analysis, were obtained (see also Supplementary Methods and Supplementary Data 1 ). Crystalline 1 was isolated by filtration, washed with MeOH (2 × 4 ml), and dried in vacuo (yield: 59%). Crystals of 1 were found to be highly hygroscopic, and always contained small amounts of water. Anal. Calc. for C 14 H 20.4 FeN 2 O 4.2 ( 1 +0.2 H 2 O): C, 49.49; H, 6.05; N, 8.24. Found: C, 49.49; H, 6.08; N, 8.27. trans -[Cu II (apH) 2 (H 2 O)] (2) A colourless MeOH solution (10 ml) of apH 2 (200 mg, 1.83 mmol) was added to 20 ml of a blue aqueous solution of Cu II (OAc) 2 ·H 2 O (184 mg, 0.92 mmol), resulting in the formation of an aqua-blue suspension after stirring the reaction mixture for 5 min. Complex 2 was isolated as an aqua-blue powder by filtration, washed with MeOH (3 × 3 ml) and Et 2 O (2 × 3 ml), before being dried in vacuo (yield: 83%). Anal. Calc. for C 12 H 14 CuN 2 O 3 ( 2 ): C, 48.40; H, 4.74; N, 9.41. Found: C, 48.13; H, 4.75; N, 9.17. Single crystals, suitable for X-ray crystallographic analysis, were obtained by layering an aqueous solution of apH 2 onto an aqueous solution of Cu II (OAc) 2 ·H 2 O (see also Supplementary Methods and Supplementary Data 2 ). Equipment for the PHERs A 200 W Hg–Xe lamp (LC8, Hamamatsu Photonics) with a quartz light guide ( Φ 5 L9588) was used as the light source. For photoirradiation at 289±10 nm, a 289 nm band pass filter (BPF) was used, while a 350 nm BPF (03 type filter) was used for irradiation at 350±10 nm. For photoirradiation at 460±10 nm, a 100 W Xe lamp (LAX-103, Asahi Spectra Co., Ltd.) with a quartz light guide ( Φ 5 × 1,000L UD0030), a VISIBLE-type mirror module and a 460 nm BPF were used. The intensity of the light was measured using a power meter (NOVA, Ophir optronics Ltd.) and a thermopile sensor (3A, Ophir optronics Ltd.). The released quantities of H 2 , HD and D 2 were measured using a gas chromatograph (GC, Shimadzu GC-2014), equipped with a 2 m column packed with either MS 5A ( T =343 K; carrier gas: Ar) or 8% KOH alumina ( T =77 K; carrier gas: He). PHER by apH 2 in MeOH A handmade Schlenk-flask-equipped quartz vessel ( V =115 ml) was charged with 1 ml of a methanolic apH 2 solution that was prepared by dissolving apH 2 (4.36 mg, 0.04 mmol) in MeOH (20 ml). Subsequently, the solution was exposed to photoirradiation in a water bath at room temperature. Gas samples (0.3 ml) were collected from the headspace of the vessel using a gas-tight syringe (Tokyo Garasu Kikai Co. Ltd.) and analysed by GC (MS 5A column). Estimated relative s.d. for H 2 (mol)/apH 2 (mol) and Φ H2 : 5%. PHER by apH − in MeOH The quartz vessel was charged with 1 ml of a methanolic apH − solution that was prepared by dissolving apH 2 (4.36 mg, 0.04 mmol) and TBAOH (10.4 mg, 0.04 mmol) in MeOH (20 ml). Subsequently, the solution was exposed to photoirradiation in a water bath at room temperature. Gas samples (0.3 ml) were collected from the headspace of the vessel using a gas-tight syringe and analysed by GC, similar to the aforementioned procedure. Estimated relative s.d. for H 2 (mol)/apH − (mol) and Φ H2 : 5%. PHER by 1 in MeOH Crystals of 1 were filtered and washed with MeOH (2 × 4 ml), before being dissolved in MeOH (4 ml) to afford a saturated pale-orange MeOH solution of 1 . Subsequently, 1 ml of this solution was transferred into the quartz vessel. The reaction and analysis were carried out as described above. Estimated relative s.d. for H 2 (mol)/ 1 (mol) and Φ H2 : 5%. Analysis of HCHO in PHER solutions An aqueous solution of AcOH (100 ml, 2.26 M) was prepared by dissolving 12.9 ml of AcOH (226 mmol) in water under an atmosphere of air. Subsequently, an aqueous solution of NH 4 OAc (200 ml, 2.25 M) was prepared by dissolving NH 4 OAc (34.68 g, 450 mmol) in water (200 ml). An AcOH/NH 4 OAc buffer solution was prepared by combining 8 ml of the aqueous AcOH solution with 200 ml of the aqueous NH 4 OAc solution. An aqueous solution (1,000 ml) of acetyl acetone and ethanol was prepared by dissolving 7 ml of acetyl acetone and 14 ml of ethanol in water (979 ml). Methanolic standard solutions of HCHO (0, 1, 5 and 10 mM) were prepared by diluting a methanolic HCHO solution (37%) with appropriate amounts of dehydrated MeOH. A mixture of the methanolic standard solutions of HCHO (0.1 ml), the AcOH/NH 4 OAc buffer solution (2.0 ml) and the aqueous acetyl acetone solution (2.0 ml) was heated to 60 °C for 15 min. Then, the solution was cooled to room temperature, and 20 μl of the reaction mixture were analysed by HPLC, using a Synergi 4u Hydro-RP80A column (Phenomenex) and H 2 O/MeCN ( v / v =85/15) at a flow rate of 1.0 ml min −1 . The targeted 3,5-diacetyl-1,4-dihydro-2,6-lutidine, which was generated from HCHO, was detected at 370 nm, and the apparent linearity of the thus obtained calibration curves suggested that a quantitative analysis of the compound in the PHER solutions should be possible ( Supplementary Fig. 4a ). To estimate the amount of HCHO produced in the PHER solutions, 0.1 ml of the corresponding reaction mixtures were used instead of the standard solutions. Estimated relative s.d. based on the calibration curves for the PHER products of HCHO: 1.4–2.5% (refs 64 , 65 , 66 , 67 , 68 ). Analysis of HCO 2 H/HCO 2 Me in the PHER solutions Methanolic standard solutions of HCO 2 H (0, 0.5, 1, 2 and 4 mM) were prepared by diluting formic acid with MeOH in water under an atmosphere of air. About 500 μl of each solution were treated with 5 μl of H 2 SO 4 at room temperature and stirred for 15 min. These HCO 2 H standard solutions were analysed by HPLC using a Synergi 4u Hydro-RP80A column and H 2 O/MeCN ( v / v =95/5) at a flow rate of 1.0 ml min −1 . Quantities of HCO 2 H/HCO 2 Me (methyl formate) were calculated based on the detected HCO 2 Me at 210 nm; given the apparent linearity of the calibration curves, a quantitative analysis of HCO 2 H/HCO 2 Me in the PHER solutions should be possible ( Supplementary Fig. 4b ). To estimate the total amount of HCO 2 H/HCO 2 Me produced in the PHER solutions, 500 μl of the corresponding reaction mixtures were used instead of standard solutions. Estimated relative s.d. based on the calibration curves for the PHER products of HCO 2 H/HCO 2 Me: 1.9–2.9% (refs 67 , 68 ). During the PHERs, HCO 2 Me may either be generated directly from MeOH, or it may be generated from the methyl-esterification of HCO 2 H with H 2 SO 4 in the presence of MeOH (HPLC pre-treatment). During the PHERs, HCO 2 H may be produced from the dehydrogenation of HCHO in the presence of trace amounts of residual H 2 O, especially in the case of apH − , which was generated in situ from the deprotonation of apH 2 by TBAOH. PHER by 1 in MeOH- d 3 All reactions and analyses were carried out as described above, except that 1 was dissolved in MeOH- d 3 , and that an 8% KOH alumina column was used for the GC analysis. The H 2 standards were detected at 5.0 ( p -H 2 ) and 6.3 min ( o -H 2 ) ( Fig. 6a ). D 2 gas was generated from the reaction of MeOH- d 4 with sodium metal, and the corresponding peaks were detected at 7.8 ( p -D 2 ) and 8.4 min ( o -D 2 ) ( Fig. 6b ). HD gas was generated from the reaction of a MeOH/MeOH- d 4 ( v / v =1/1) mixture with sodium metal, and the corresponding signals for HD were detected at 6.4 min ( Fig. 6c ). Since pure HD gas was unobtainable, the calibration and quantitative estimation of generated HD could not be carried out. PHER by apH 2 and 1 in the presence of scavengers All reactions were carried out as described above for the PHER procedures, except for using a quartz NMR tube as the reaction vessel and MeOH- d 4 as the solvent. For that purpose, apH 2 or 1 were dissolved in degassed MeOH- d 4 (apH 2 : 2 mM; 1 : 1 mM) with t -BuSH or NADCl (2 mM), before the solutions were analysed by 1 H NMR spectroscopy prior and posterior to photochemical reactions. Physical measurements 1 H NMR (500 MHz) spectra were measured on a JEOL EX-500 spectrometer. Elemental analyses were carried out on a Perkin-Elmer 2400 II CHN analyzer. Ultraviolet–visible–near infrared spectra (200–3,300 nm) in solution or in the solid state (KBr pellets) were recorded on a Hitachi U-4100 spectrophotometer at 296 K. HPLC measurements were carried out on a Shimadzu LC-20AT liquid chromatograph, equipped with an SPD-20A ultraviolet–visible detector. Emission spectra were recorded on a Horiba fluoromax using MeOH solutions of apH 2 and 1 at 296 K. Calculations of external quantum yields ( Φ H2 ) MeOH solutions of apH 2 , apH − and 1 were irradiated at 289±10 or 350±10 nm. The amount of H 2 evolved during the subsequent 5 h was used to calculate the Φ H2 according to the following equations: wherein, N H2 , N p , E I , E p , R , M H2 , N A , I , t , h , c and A refer to the number of molecules of evolved H 2 per mol of catalyst, the number of absorbed photons, the energy of the irradiation source, the energy of the irradiation photons, the proportion of the catalyst that is absorbing light, the mol number of the evolved H 2 , the Avogadro constant, the optical intensity of the light, the irradiation time, the Planck constant, the speed of light in vacuum and the absorbance of the catalyst in MeOH, respectively. The absorbance throughout the photoreaction was assumed to be constant at an optical length of 1.0 cm: apH 2 (5.72 at 289 nm), apH − (5.39 at 289 nm) and 1 (7.76 at 289 nm, 1.15 at 350 nm). Data availability The data supporting the results of this study are available from the article and its Supplementary Information file, or from the authors upon request. The X-ray crystallographic coordinates used for the structure determination reported in this article have been deposited at the Cambridge Crystallographic Data Centre (CCDC) under deposition numbers CCDC-1062112 ( 1 ) and CCDC-1418535 ( 2 ). These data can be obtained free of charge from The Cambridge Crystallographic Data Centre via www.ccdc.cam.ac.uk/data_request/cif . How to cite this article: Wakizaka, M. et al . Dehydrogenation of anhydrous methanol at room temperature by o -aminophenol-based photocatalysts. Nat. Commun. 7:12333 doi: 10.1038/ncomms12333 (2016).